Nondispersive optical activity of meshed helical metamaterials Extreme optical properties can be realized by the strong resonant response of metamaterials consisting of subwavelength-scale metallic resonators. However, highly dispersive optical properties resulting from strong resonances have impeded the broadband operation required for frequency-independent optical components or devices. Here we demonstrate that strong, flat broadband optical activity with high transparency can be obtained with meshed helical metamaterials in which metallic helical structures are networked and arranged to have fourfold rotational symmetry around the propagation axis. This nondispersive optical activity originates from the Drude-like response as well as the fourfold rotational symmetry of the meshed helical metamaterials. The theoretical concept is validated in a microwave experiment in which flat broadband optical activity with a designed magnitude of 45° per layer of metamaterial is measured. The broadband capabilities of chiral metamaterials may provide opportunities in the design of various broadband optical systems and applications. Polarization is one of the most fundamental and important aspects of electromagnetic waves. The manipulation of the polarization state is crucial in the design and realization of various optical systems because the electromagnetic response of a material or a device generally depends on the polarization states of incident electromagnetic waves. Traditionally, manipulation of polarization states has been achieved by the use of wave plates, gratings [1] , prismatic rotators [2] or natural chiral media [3] . Compared with other devices, chiral media have an intrinsic benefit of requiring no rotational adjustment; the rotational state of the chiral media around their own optical axis does not affect the optical rotatory power. The term ‘chiral’ refers to the structural characteristic of an object that lacks any mirror symmetries. In chiral media, electric and magnetic fields are cross-coupled, so that the degeneracy between right and left circularly polarized waves (RCP and LCP waves) is lifted. This broken degeneracy results in nonidentical refractive indices for the RCP and LCP waves. As a result, the polarization plane of a linearly polarized, electromagnetic wave travelling in chiral media is rotated, and this phenomenon is called optical activity. However, the strength of optical activity in natural chiral media is small and dispersive, thus rendering broadband polarization rotation inefficient with natural chiral media. In recent years, chiral media that possess strong chirality have been constructed artificially. Much attention has been focused on their potential route to negative refraction/reflection [4] , [5] , [6] , [7] , [8] , [9] , [10] , [11] , [12] , asymmetric transmission [13] , [14] , [15] , [16] , [17] and the observation of repulsive Casimir force [18] , [19] , as well as their gigantic optical activity and circular dichroism [8] , [9] , [12] , [20] , [21] , [22] , [23] , [24] , [25] , [26] , [27] , [28] , [29] , [30] . Utilizing strongly resonant, chiral meta-molecules, the limitation of weak optical activity can be overcome. Yet, despite unnaturally strong chirality of resonant-type chiral metamaterials, highly dispersive optical activity and corresponding narrow transmission bandwidth still were hampering the achievement of broadband polarization manipulation [7] , [9] , [12] , [20] , [21] , [26] . Recently, there have been a few attempts to achieve nondispersive optical activity with metamaterials based on complementary configurations; however, the intrinsic resonant properties of the meta-atoms that were used still limited the operating bandwidth [31] , [32] . Furthermore, two characteristic optical properties of chiral media, that is, circular birefringence and dichroism, coexist in the operating frequency band so that the realization of pure broadband optical activity is a critical and current issue for chiral metamaterials. In the presence of significant circular dichroism, a linearly polarized wave travelling through chiral metamaterials becomes elliptically polarized, which exemplifies the inadequacy of resonant chiral metamaterials as polarization rotators. Here we demonstrate that extremely broadband, nondispersive, strong optical activity with high transparency can be obtained with nonresonant, meshed helical metamaterials (MHMs). This nonresonant behaviour of MHMs comes from their Drude-like response that results in 1/ ω dispersion of effective chirality parameter κ . Furthermore, it is shown that circular dichroism is essentially absent in a wide range of operating frequencies. In contrast to other work based on an array of helices with parallel configuration [24] , [33] , [34] , [35] , [36] , [37] , [38] or metallic gyroid structures with mixtures of right- and left-handed helices [39] , [40] , the double-helix structures in MHMs are networked and arranged with fourfold rotational symmetry around the wave propagation axis. To prove the nondispersive, strong optical activity of MHMs, samples designed to rotate the polarization state by 45° per layer are fabricated and measured. The optical rotary power of a single-layer MHM can be engineered by varying the thickness of the MHM wires, and the optical activity of the stacked MHMs can be made proportional to the number of layers. It also is found that the transmission bandwidth can be easily tailored by varying the interlayer spacing. Unit cell of MHMs An MHM can be configured with double helical metallic structures as its building blocks ( Fig. 1a ). Within the MHM, the helices are arranged densely with fourfold rotational symmetry along the wave propagation axis. The rotational symmetry of metallic helical structures in MHMs leads to the nondispersive optical activity and extinction of circular dichroism. Furthermore, by utilizing the double helix as a building block rather than a single helix, the magnitude of optical activity can be enhanced in MHMs, similar to the case of parallel configuration of helical structures, where the circular dichroism is enhanced with double helix arrays [41] , [42] , [43] . The rotational symmetry of the unit cell assures the eigenpolarizations for MHMs under normal incidence to be a pair of circular polarizations [44] , which results in invariant optical properties for arbitrary input polarization angles. With the excitation of electromagnetic waves on MHMs, magnetic and electric dipole moments are induced in the transverse direction of the axis of wave propagation ( Fig. 1a ). These dipole moments can be excited by either an electric filed or a magnetic field parallel to the helical axis of each helix in the MHM. 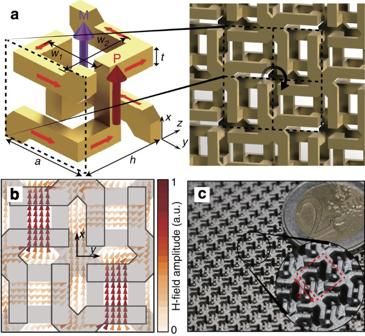Figure 1: Basic concepts. (a) Schematic illustration of MHM. The unit cell is composed of four double-helix metallic structures (left side of the figure), densely arranged with fourfold rotational symmetry around thezaxis that assures the incident polarization-independent property. The incident electric fieldEinduces the surface current and electric dipole momentP. The current excites the strong magnetic dipole momentMalong the parallel direction ofP. (b) The numerically calculatedHfield distribution atz=−h/2 plane of unit cell (at 7.2 GHz) is shown with impinging electric field polarized in the direction of thexaxis. (c) Photograph of the fabricated sample of MHM. The size of the fabricated sample was 170 × 170 mm. The lattice constant of the primitive unit cell (indicated as a red dashed square) is represented asα=3.66 mm. Samples with the following structural dimensions were tested:a=2.59 mm,w1=1.15 mm,w2=2.0 mm,t=0.50 mm andh=2.5 mm. Figure 1b shows the magnetic field distribution in the plane of z =− h /2 when the incident electric field is polarized in the x direction, which clearly shows that the magnetic dipole moment is induced strongly along the parallel direction to the electric field of the incident wave. This strong magnetoelectric coupling leads to the large optical activity of MHMs. Figure 1c shows a photographic image of an MHM fabricated with acrylic resin and silver by commercial, layered-prototyping equipment. Utilizing a pair of linearly polarized, broadband horn antennas, the chiral properties of MHMs are characterized in microwave frequencies (see Methods). Figure 1: Basic concepts. ( a ) Schematic illustration of MHM. The unit cell is composed of four double-helix metallic structures (left side of the figure), densely arranged with fourfold rotational symmetry around the z axis that assures the incident polarization-independent property. The incident electric field E induces the surface current and electric dipole moment P . The current excites the strong magnetic dipole moment M along the parallel direction of P . ( b ) The numerically calculated H field distribution at z =− h /2 plane of unit cell (at 7.2 GHz) is shown with impinging electric field polarized in the direction of the x axis. ( c ) Photograph of the fabricated sample of MHM. The size of the fabricated sample was 170 × 170 mm. The lattice constant of the primitive unit cell (indicated as a red dashed square) is represented as α =3.66 mm. Samples with the following structural dimensions were tested: a= 2.59 mm, w 1 =1.15 mm, w 2 =2.0 mm, t =0.50 mm and h =2.5 mm. Full size image Nondispersive optical activity The simulated and measured total transmission amplitudes, defined as for a single-layer MHM, are plotted in Fig. 2a . The total transmission approaches nearly unity at 7.2 GHz, corresponding to the impedance-matching frequency to free space ( Supplementary Fig. 1 ). 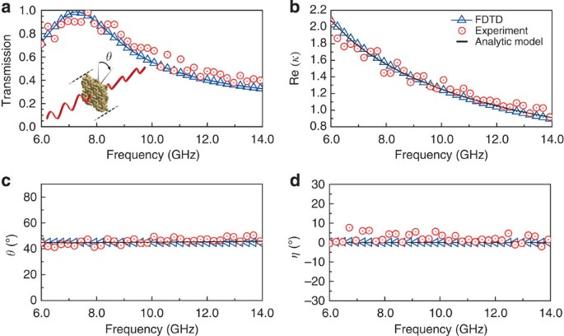Figure 2: Characterization of a single-layer MHM in the microwave range. (a) Numerically calculated and experimentally measured total transmission amplitude defined asis shown. (b) Numerically- and experimentally retrieved chirality parameterκfitted to the analytic model. (c) Nondispersive polarization rotation and (d) nearly-zero ellipticity are shown. Figure 2b shows the retrieved chirality parameter from the measurement and that calculated from a finite-difference time-domain (FDTD) simulation. It can be seen clearly that the real part of chirality parameter κ is proportional to 1/ ω . The real part and the imaginary part of κ are related to the magnitude of circular birefringence and dichroism, respectively. The inverse proportionality of the real part of the chirality parameter to the frequency leads to the broadband and nondispersive optical activity ( Fig. 2c ), since the polarization rotation θ can be explicitly expressed as θ =Re( κ )· ωh / c 0 . From numerical calculations, the upper bound in the frequency range of the nearly nondispersive optical activity reaches ~42 GHz, at which a higher mode starts to dominate ( Supplementary Fig. 2 ). Moreover, the ellipticity η is nearly zero over all measured frequency ranges, and, therefore, the polarization state of the transmitted wave still remains linearly polarized ( Fig. 2d ). It can be seen that all experimental results and simulations are in very good agreement. Figure 2: Characterization of a single-layer MHM in the microwave range. ( a ) Numerically calculated and experimentally measured total transmission amplitude defined as is shown. ( b ) Numerically- and experimentally retrieved chirality parameter κ fitted to the analytic model. ( c ) Nondispersive polarization rotation and ( d ) nearly-zero ellipticity are shown. Full size image Drude-like response of MHMs The nondispersive behaviour of optical activity can be attributed to the Drude-like response of MHMs. In general, resonant-type chiral metamaterials, for which the current distribution is localized in the unit cell, have distinct Lorentz-like electric and magnetic resonances, and the dispersive optical activity becomes inevitable near these resonance frequencies [9] , [19] , [21] , [26] , [27] , [45] . However, in the unit cell of the proposed MHM, four double-helix structures were interconnected so that the current flows freely through the metallic helix network with Drude-like behaviour. For an intuitive understanding of the nonresonant behaviour of MHMs, we developed an effective circuit model in which the double-helix structure in Fig. 1a (constituting a quadrant of the unit cell) was assumed to have total lumped inductance L and resistance R . Under electromagnetic excitation, the average electric displacement and magnetic flux density for a single-layer MHM can be derived as follows (see Methods): where S is the cross-sectional area of a double helix, V 0 is the volume of a unit cell and γ is the dissipation constant, defined as R/L . In correspondence with the constitutive equation of general chiral media with reciprocity, the effective chirality parameter of MHM can be estimated as: Assuming negligible dissipation with a substrate-free metallic network at microwave frequencies, the chirality parameter assumes a real value, which results in an inverse proportionality between the chirality parameter and the frequency. This scaling law of the chirality parameter can be confirmed by numerical simulation and measurement ( Fig. 2b–d ). It is worthwhile noting that the imaginary part of κ in the transmission band is very small, even in the presence of significant dissipation because it decays very rapidly with ω −2 so that the real part of κ is dominant in the transmission band. Therefore, little circular dichroism exists for the transmitted waves, and, thus, linearly polarized input waves maintain their polarization states in MHMs. Scaling of optical activity with a geometrical parameter For proof of the concept with an experimental demonstration, the geometrical parameters of the MHMs were chosen specifically such that the polarization rotation was 45° for a single-layer MHM. However, optical rotary power can be tuned easily by varying the thickness t of the wire of the structure ( Fig. 1a ). 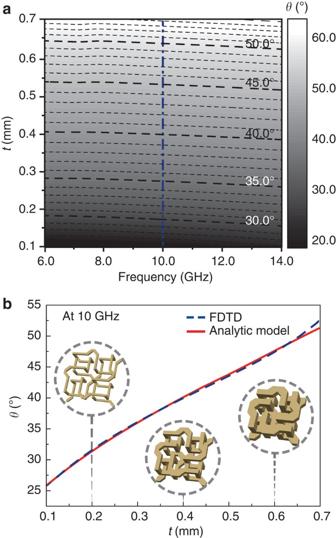Figure 3: Width-dependent broadband optical activity of a single-layer MHM. (a) Numerically calculated polarization rotation angle through a single-layer MHM depending on the thickness of the wiretof the helical structures with iso-angle lines (black dashed lines). The rotation angle is increased with the thickness of the wire, while the nondispersive property of optical activity was barely affected. (b) Simulated polarization rotation with varyingtplotted at 10 GHz and fitted with the analytical model; the following fitting parameters were used:K1=0.331 andK2=3.384. Figure 3a shows the simulated polarization rotation for a single-layer MHM with variation in t , where the optical activity was found to be correlated strongly with the thickness of the wire. As can be seen in the plot, the optical activity becomes stronger with increasing t , while the nondispersive property still is preserved. In order to clearly show this scaling behaviour, the optical activity at 10 GHz was plotted in Fig. 3b as a function of t . This behaviour can be predicted by the analytical model with the lumped inductance L of a double helix approximated by (refs 33 , 46 ). Here K 1 and K 2 are structural fitting parameters that are dependent on the shapes of the inductors, t is the thickness of the wire and w is the effective mean diameter of the helices given by , which was introduced to simplify the equation ( Fig. 1a ). Substituting this inductance formula into equation (2), the expression for the polarization rotation after travelling a single-layer MHM can be written as: Figure 3: Width-dependent broadband optical activity of a single-layer MHM. ( a ) Numerically calculated polarization rotation angle through a single-layer MHM depending on the thickness of the wire t of the helical structures with iso-angle lines (black dashed lines). The rotation angle is increased with the thickness of the wire, while the nondispersive property of optical activity was barely affected. ( b ) Simulated polarization rotation with varying t plotted at 10 GHz and fitted with the analytical model; the following fitting parameters were used: K 1 =0.331 and K 2 =3.384. Full size image This scaling behaviour is plotted in Fig. 3b , and it fits well with the numerical simulation. Tailoring the transmission bandwidth of MHMs In general, the effective parameters of bulk metamaterials are different from those of a constituting metamaterial layer in the presence of strong interlayer coupling [7] , [9] , [21] , [23] , [27] , [45] , [47] , [48] . However, interlayer coupling between MHMs is negligibly small because the magnetic field in MHMs is highly localized inside the helices, as can be seen in Fig. 1b . Therefore, a single-layer MHM can be considered as a homogeneous thin film, and the transmission coefficients for stratified MHMs can be calculated by the characteristic matrix formalism [49] , [50] . With a numerically obtained matrix for a single-layer MHM, the transmission through double-layered MHMs with different interlayer spacing distances can be calculated as shown in Fig. 4a . The results from FDTD simulations also are plotted along with those from the characteristic matrix method in Fig. 4a and compared with the experimental data. In the measurements, we inserted polyethylene plates with three thicknesses, that is, s =1.5, 3.0 and 5.0 mm to certify the exact distance between the two layers. The agreement between the characteristic matrix method, FDTD simulation and experimental data confirmed the negligibly small interlayer coupling in MHMs. Unlike in previous single-layer measurements, two transmission peaks were observed for the double-layered MHM. Notably, by narrowing the interlayer spacing, the frequency difference between two distinct transmission peaks increased, and the transmission band widened. The number of transmission peaks is equal to the number of stacked MHM layers; the transmission peaks (except for the lowest frequency one) originate from the Fabry–Pérot resonances of the multilayered metamaterial slab ( Supplementary Fig. 3 ). It can be predicted that a spectral transmission band will be formed by increasing the number of layers and that the corresponding transmission bandwidth will be determined directly by the interlayer spacing ( Fig. 5 ). As can be seen for the measured and calculated range of spacing distances in Figs 4 and 5 , the magnitude of optical activity is barely affected by the spacing distance because of negligible interlayer coupling. By stacking more layers, the polarization rotation can be increased linearly; for example, 135° for three layers and 180° for four layers. This spacing-independent optical activity is very desirable for manipulating the polarization because we could tailor the transmission bandwidth by varying the spacing without considering the interlayer effect on the magnitude of optical activity. 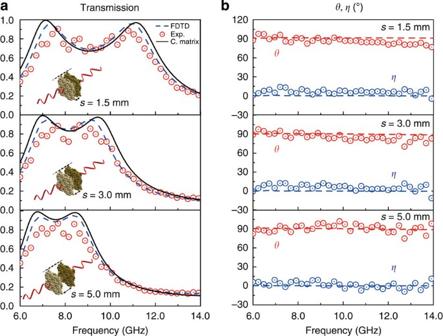Figure 4: Tailoring transmission bandwidth of double-layered MHMs. (a) Total transmission spectra for double-layered MHM, showing the results of experiments, FDTD simulation and the characteristic matrix method with different values of interlayer spacings. (b) Corresponding polarization rotation and ellipticity with varyings.The red and blue dashed lines represent simulated polarization and ellipticity, respectively. The circles represent the corresponding experimental data. The following dimensions of interlayer spacing were tested:s=1.5, 3.0 and 5.0 mm. Figure 4: Tailoring transmission bandwidth of double-layered MHMs. ( a ) Total transmission spectra for double-layered MHM, showing the results of experiments, FDTD simulation and the characteristic matrix method with different values of interlayer spacing s . ( b ) Corresponding polarization rotation and ellipticity with varying s. The red and blue dashed lines represent simulated polarization and ellipticity, respectively. The circles represent the corresponding experimental data. The following dimensions of interlayer spacing were tested: s =1.5, 3.0 and 5.0 mm. 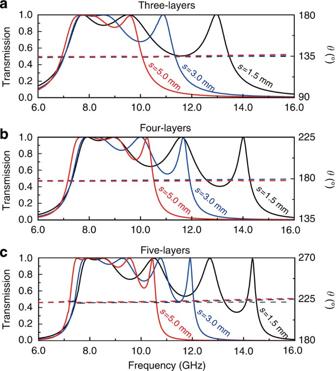Figure 5: Total transmission and polarization rotation for multilayered MHMs. Numerically calculated total transmission and polarization rotation as a function of the interlayer spacing for (a) three-layer-, (b) four-layer- and (c) five-layer MHMs. The solid and dashed lines represent the transmission spectra and polarization rotations, respectively. The metal was assumed to be a perfect electric conductor and no spacer was assumed to be inserted between the layers. Full size image Figure 5: Total transmission and polarization rotation for multilayered MHMs. Numerically calculated total transmission and polarization rotation as a function of the interlayer spacing for ( a ) three-layer-, ( b ) four-layer- and ( c ) five-layer MHMs. The solid and dashed lines represent the transmission spectra and polarization rotations, respectively. The metal was assumed to be a perfect electric conductor and no spacer was assumed to be inserted between the layers. Full size image We have shown that nondispersive optical activity can be realized with MHMs. This nonresonant property originates from the Drude-like response of MHMs. Since the thickness of a single-layer MHM is much smaller than the operating wavelength, MHMs can be utilized for broadband and ultrathin polarization manipulators. With the scaling behaviour of optical rotary power with respect to the thickness of the wire, the polarization rotation can be manipulated very easily, even with a single-layer MHM. Furthermore, the polarization rotation can be increased in proportion to the number of MHM layers, and the transmission bandwidth can be tailored by varying the interlayer spacing between the MHM layers. The proposed concept was validated experimentally in the microwave range; however, it is worth pointing out that the operating frequency could be shifted to a higher band by adjusting the size of the unit cell; for example, by utilizing modern nano/micro fabrication techniques such as direct laser writing [24] , [51] , MHMs that operate in the terahertz or far-infrared frequency ranges might be fabricated. Sample fabrication The supporting structure of the MHM was fabricated with an acrylic resin (EX200, 3D Systems) with commercial, layered-prototyping equipment (ProJet3000, 3D Systems) and coated with silver paste (P-100, Elcoat) for its metallic properties. The lateral dimensions of the structure were 170 × 170 mm. Analytic descriptions for effective parameters To qualitatively understand the frequency- and geometry-dependent effective parameters of MHMs, we calculate the induced polarization and magnetization resulting from the excitation of electromagnetic waves. For the sake of simplicity, the double helix structures that constituted the quadrants of the unit cell are assumed to be modelled with lumped inductance L and resistance R . In homogeneous electric and magnetic fields, the electric potential U is given by: where S is the cross-sectional area of the helices defined as S = w 1 w 2 . Applying the effective RL circuit model, we have: where the ± signs correspond to right- and left-handed double helix structure and I w is the total current that flows through the metallic helices. Assuming the solution is time-harmonic, the formula for the total current can be obtained as: From equation (6), the effective electric and magnetic dipole moments can be derived as follows: where V 0 is the volume of a unit cell and γ is the dissipation constant defined as R/L. Noting that D = ε 0 E + P , B = μ 0 H + μ 0 M and that the unit cell of MHM has a fourfold rotational symmetry, the average electric displacement and magnetic flux density under normal incidence can be derived as follows: From equation (8) and the constitutive equation of general chiral media with reciprocity, the effective parameters of MHM can be assigned as follows: where ε b and μ b are added for quantitative fitting of effective parameters ( Supplementary Fig. 4 ). Characterization of optical activity The experiment was conducted with linearly polarized, broadband horn antennas and a network analyser to measure the scattering parameters. To characterize the MHM, polarization rotation and circular dichroism were estimated from the scattering parameters that were measured [52] . The magnitude of polarization rotation was calculated as , where T is the complex transmission for the RCP (LCP) wave derived from co-polarized ( T xx ) and cross-polarized ( T yx ) transmission coefficients, T ± = T xx ± iT yx . Circular dichroism can be characterized with the ellipticity . In addition, the effective chirality parameter κ can be obtained as and , where h is the thickness of the sample. How to cite this article: Park, H. S. et al . Nondispersive optical activity of meshed helical metamaterials. Nat. Commun. 5:5435 doi: 10.1038/ncomms6435 (2014).